Designing a robustly metallic noncenstrosymmetric ruthenate oxide with large thermopower anisotropy The existence of ~30 noncentrosymmetric metals (NCSM) suggests a contraindication between crystal structures without inversion symmetry and metallic behaviour. Those containing oxygen are especially scarce. Here we propose and demonstrate a design framework to remedy this property disparity and accelerate NCSM oxide discovery. The primary ingredient relies on the removal of inversion symmetry through displacements of atoms whose electronic degrees of freedom are decoupled from the states at the Fermi level. Density functional theory calculations validate this crystal-chemistry strategy, and we predict a new polar ruthenate exhibiting robust metallicity. We demonstrate that the electronic structure is unaffected by the inclusion of spin–orbit interactions, and that cation-ordered SrCaRu 2 O 6 exhibits a large thermopower anisotropy (|Δ S ⊥ |~6.3 μ V K −1 at 300 K) derived from its polar structure. Our findings provide chemical and structural selection guidelines to aid in the search of NCSM with enhanced thermopower anisotropy. The metallic features in materials, which provide low-resistance channels for electrical conduction, lead to effective screening of local electric dipole moments [1] . Itinerant electrons disfavour both their formation and cooperative ordering [2] . In spite of the incompatibility between acentricity and metallicity, metallic materials that break the spatial parity operation mapping were originally discussed in the 1960s by Matthias and then, later more rigorously by Anderson and Blount [3] . The first experimental identification [4] of a candidate polar metal, the binary intermetallic V 2 Hf, was made a decade later. Since then, more noncentrosymmetric metals (NCSM) have been identified ( Fig. 1 ) and found to exhibit unconventional optical responses [5] , [6] , magnetoelectricity [7] , [8] and superconductivity [9] , [10] , [11] . Yet, they remain challenging to discover. The principal NCSM material classes are binary and ternary intermetallics and silicides. Intriguingly, few NCSM are oxides with the notable exceptions [12] , [13] , [14] , [15] of a layered cuprate (Y 1− x Ca x Sr 2 GaCu 2 O 7± y ), a geometrically frustrated pyrochlore (Cd 2 Re 2 O 7 ), and recently LiOsO 3 with a structural transition similar to ferroelectric LiNbO 3 . (Degenerately doped dielectrics like BaTiO 3− δ (ref. 16 ) and ZnO:Al [17] , although exhibiting metallic resistivity, are not intrinsically metallic and NCS—their conductivity is high because of deviations from ideal stoichiometry.) 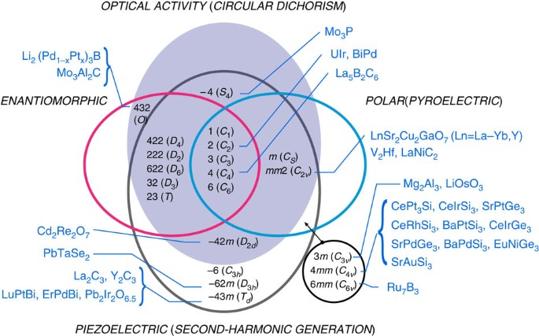Figure 1: Classification of noncentrosymmetric metals. Known compounds differentiated by crystal class following the NCS classification scheme introduced in Halasyamani and Poeppelmeier65include 4dand 5dtransition metal intermetallics, carbides or silicides. Oxide compounds are scarce. Figure 1 suggests that NCSM tend to require cations with large atomic masses, but this is not always the case, for example, Mg 2 Al 3 . The absence of reliable crystal-chemistry guidelines and the limited understanding of the microscopic origin of inversion symmetry-lifting displacements in metals poses a serious challenge for their discovery: how does one explain, let alone design, cooperative acentric atomic displacements in crystalline oxide conductors? Figure 1: Classification of noncentrosymmetric metals. Known compounds differentiated by crystal class following the NCS classification scheme introduced in Halasyamani and Poeppelmeier [65] include 4 d and 5 d transition metal intermetallics, carbides or silicides. Oxide compounds are scarce. Full size image In this work, we present a microscopic understanding for NCSM, leading to a design principle that we use in the theoretical prediction of a polar NCSM transition metal (M) oxide. We formulate a two-step material selection process based on a weak electron–lattice coupling principle that considers the symmetry and atomic species participating in the inversion-lifting lattice modes, and the susceptibility of the cations’ electronic configurations to a metallic state. We show that two k ≠0 lattice modes describing rotations of MO 6 octahedra induce polar A-cation displacements in the layered and cation-ordered (Sr,Ca)Ru 2 O 6 perovskite, for which experimental solid solutions [18] are metallic. Because the microscopic mechanism is independent of the details of the states at the Fermi level, unlike conventional dipolar interactions that are essential to stabilizing acentric displacements of second-order Jahn–Teller cations in dielectrics [19] , the design strategy is readily transferable to other transition metal chemistries. We show that spin–orbit interactions (SOI) do not alter the electronic ground state, and that the unusual coexistence of a polar axis and metallicity produces a novel correlated material possessing a highly anisotropic thermopower response (|Δ S ⊥ |~6.3 μ V K −1 at 300 K) with nearly isotropic electrical conductivity. Design of a metallic oxide without inversion Our design strategy originates from Anderson’s work [3] on ‘ferroelectric metals,’ where he writes that “while free electrons screen out the electric field [in materials] completely, they do not interact very strongly with the transverse optical phonons and the Lorentz local fields [that] lead to ferroelectricity, since umklapp processes are forbidden as k →0.” We recast this observation into an operational principle that states: the existence of any NCSM relies on weak coupling between the electrons at the Fermi level, and the (soft) phonon(s) responsible for removing inversion symmetry. An essential, implicit, materials constraint is that the low-energy electronic structure derives from an electron count giving partial band occupation, which may be obtained by judicious selection of the cation chemistries. We identify three displacive routes fulfilling the weak-coupling hypothesis in solid-state systems, specified by the symmetry behaviour of the lattice phonons that would remove inversion symmetry in a centrosymmetric metal and yield a NCS crystal structure ( Table 1 ). It should be noted that an order–disorder mechanism could also be operative; the classification of such symmetry breaking is consistent with our scheme; the caveat being that the soft phonon is replaced by an order parameter that describes atomic site occupancy. In either case the same set of irreducible representations may be used. Table 1 Routes to lift inversion symmetry in metallic compounds. Full size table The third approach, which we focus on here, resembles a condition that supports a novel ‘improper’ mechanism [20] , [21] for ferroelectricity that has been exploited to design artificial polar oxides with sizeable electric polarizations by heterostructuring non-polar dielectrics. Note that throughout we choose to refer to these materials as NCS metals rather than ‘ferrroelectric metals’ as articulated by Anderson and recently others to eliminate misconceptions about the presence of switchable spontaneous electric polarizations in metals, and more accurately describe the crystallographic–electronic function of the materials. In this way, one can generally and completely classify all metals without inversion symmetry and not solely those of the polar subset of NCS structures ( Fig. 1 ). Within this framework, the design of a NCSM oxide using geometric-induced displacements requires an oxide class exhibiting coupled zone-boundary phonons that lift inversion symmetry. Here we choose orthorhombic AMO 3 perovskites with corner-connected MO 6 octahedra that are rotated about each Cartesian axis; the ‘tilt’ pattern is obtained and described by two phonons with k =(½, ½, 0) and (½, ½, ½) wavevectors relative to the cubic aristotype [22] . The a + b − c − MO 6 rotation pattern in the presence of layered A-cation order along a [001] direction, for example, accessible through synthetic bulk chemistry routes [23] , [24] or heteroepitaxial thin-film growth methods [25] , is sufficient to produce a polar structure [26] , [27] . The chemical species are selected given the constraints that the rotations of octahedra are necessary—determined by the A and M cation size mismatch in perovskites—and that the electronic configuration of the M cation results in a nonzero density-of-states at the Fermi level ( E F ). These requirements should be satisfied for ordered (Sr,Ca)Ru 2 O 6 , since both bulk SrRuO 3 and CaRuO 3 are experimentally found in the a + b − c − Glazer tilt pattern and also have partially occupied low-energy Ru 4 d t 2 g orbitals. 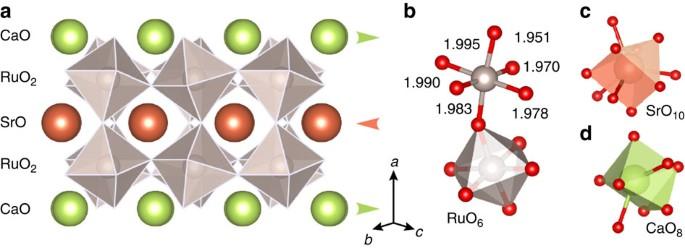Figure 2: Ground state structure of the polar noncentrosymmetric metal (Sr,Ca)Ru2O6. Crystal structure of cation-ordered (Sr,Ca)Ru2O6with thea+b−b−RuO6tilt pattern (a). The off-centre Ru4+distortions (bond lengths in Å) produce local dipoles that cooperatively order along thecdirection (b), removing the mirror plane perpendicular to the A-site cation order. The local coordination environment for (c) Sr (tetra-capped trigonal prism) and (d) Ca (bi-capped trigonal prism) reveals that large A-site distortions from the ideal 12-fold coordination occur in opposite directions (arrows), along the polarcaxis. Ground-state structure Figure 2 depicts the polar Pmc 2 1 ground state crystal structure of (Sr,Ca)Ru 2 O 6 obtained from density functional theory calculations. (See Supplementary Table 1 for the crystallographic data.) The extended RuO 6 structure is highly rotated, adopting the targeted orthorhombic tilt pattern with rotations of adjacent octahedra out-of-phase about the [011] direction and in-phase about the layering [100] direction ( Fig. 2a ). The Ru–O–Ru bond angles are 157.1° and 145.6° (perpendicular to the CaO/SrO layers) and 150.4° (within the layers). The stabilization of this rotation pattern is understood on the grounds that the π* band, which is nearly full because of the configuration, is shifted to lower energy by the electronegative Ru 4+ cation [28] . Figure 2: Ground state structure of the polar noncentrosymmetric metal (Sr,Ca)Ru 2 O 6 . Crystal structure of cation-ordered (Sr,Ca)Ru 2 O 6 with the a + b − b − RuO 6 tilt pattern ( a ). The off-centre Ru 4+ distortions (bond lengths in Å) produce local dipoles that cooperatively order along the c direction ( b ), removing the mirror plane perpendicular to the A-site cation order. The local coordination environment for ( c ) Sr (tetra-capped trigonal prism) and ( d ) Ca (bi-capped trigonal prism) reveals that large A-site distortions from the ideal 12-fold coordination occur in opposite directions (arrows), along the polar c axis. Full size image (Sr,Ca)Ru 2 O 6 exhibits small off-centre Ru distortions ( Fig. 2b ) and large A-site cation displacements ( Fig. 2c,d ). Acentric B-site displacements are common to TMs with d 0 -electronic configurations in octahedral coordinations; however, for d n , n ≥1, such polar displacements are largely disfavoured, that is, the energetic gain due to d π− p π metal–oxygen bonding decreases on filling the t 2 g orbital [29] . Nonetheless, we find they occur for d 4 Ru 4+ , displacing the metal centre nearly towards an edge (~0.03 Å), staying in the (110) plane (see Supplementary Table 2 ). This results in one short, two long and three medium Ru–O bonds ( Fig. 2b ), which are close to the average value found experimentally in the Sr 0.5 Ca 0.5 Ru 2 O 3 solid solution [30] . 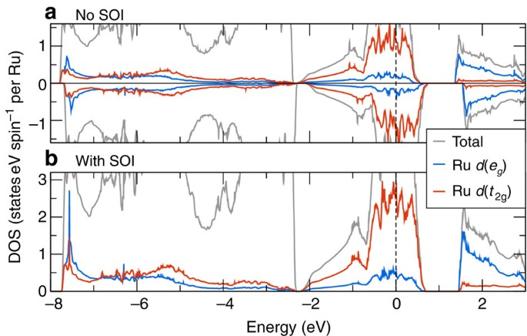Figure 3: Electronic structure. The total (black line) and Ru 4dorbital- and spin-resolved densities of states (DOS) of orthorhombic (Sr,Ca)Ru2O6calculated (a) without spin–orbit interactions (SOI) and (b) with SOI. The Fermi level is at 0 eV (dashed line). The Ca and Sr atoms make large polar displacements (0.29 and 0.21 Å, respectively) along the [001] and [ ] directions (see Supplementary Table 3 ), resulting in distorted polyhedra ( Fig. 2c ). We explore these displacements and their effect on the electronic structure in more detail below. Electronic properties Figure 3 shows the total and partial densities-of-states (DOS) for the polar NCSM (Sr,Ca)Ru 2 O 6 without ( Fig. 3a ) and with ( Fig. 3b ) SOI. The valence band is composed largely of O 2 p states hybridized with Ru 4 d states, with the oxygen states predominately found in regions below the E F . Consistent with low-spin Ru 4+ , the large peaks in the DOS near E F are caused by the fairly flat Ru t 2 g bands, whereas the strongly hybridized e g orbitals form broader bands in the conduction band beginning near 1.5 eV. We find that without SOI, weakly dispersive t 2 g bands lead to a large number of states at the Fermi level, that is, N ( E F )~2.2 eV per spin per Ru atom indicating robust metallic behaviour ( Fig. 3a ), despite a ~0.75 eV band gap present in both spin channels far above E F (0.5 eV). It is also ferromagnetic (0.914 μ B f.u. −1 ) with ~0.35 μ B per Ru atom; the remaining magnetization is distributed among the oxygen ligands due to the itinerant spin-polarized electrons. Using a simple modified Weiss formula [31] , we calculate a Curie temperature T c =47 K (27 K applying Anderson’s rescaling [32] ) in good agreement with experimental data [18] on solid solution Sr 0.5 Ca 0.5 RuO 3 ( T c =57 K). Figure 3: Electronic structure. The total (black line) and Ru 4 d orbital- and spin-resolved densities of states (DOS) of orthorhombic (Sr,Ca)Ru 2 O 6 calculated ( a ) without spin–orbit interactions (SOI) and ( b ) with SOI. The Fermi level is at 0 eV (dashed line). Full size image Since SOI play a significant role in determining the orbital structure in 3 d transition metal oxides [33] , [34] , we calculate the DOS with SOI ( Fig. 3b ). Although the SOI enable the spin-up and spin-down bands to mix, we find an electronic structure similar to that without the interactions. The Ru 4 d -band occupation at E F is weakly modified and the gap in the conduction band is slightly reduced. Nonetheless, the weakly dispersed t 2 g states persist, and (Sr,Ca)Ru 2 O 6 remains metallic [ N ( E F )~4.36 eV per Ru atom] consistent with SOI calculations on bulk SrRuO 3 (ref. 35 ), where spin–orbit coupling also does not greatly alter the electronic structure. Origin of acentricity For purposes of evaluating the design approach and the proposed geometric-induced inversion symmetry-breaking displacements, we perform a group theoretical analysis [36] , [37] of the Pmc 2 1 structure with respect to a fictitious prototypical centrosymmetric phase ( P 4/ mmm symmetry), reducing the polar structure into a set of symmetry-adapted modes associated with different irreducible representations of the P 4/ mmm phase (see Supplementary Fig. 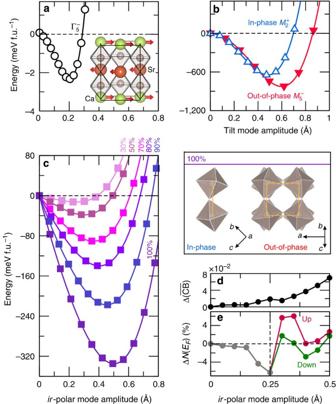Figure 4: Electron–lattice interactions on the ground state stability. (a) Polar (ir-active) mode withsymmetry. The inset depicts the polar cation displacement pattern; apical oxygen and (small) Ru displacements are omitted for clarity. (b) In-phase and out-of-phase RuO6rotational modes. (c) Normalized energy gain obtained by increasing amplitude of the polar displacements at fixed percentages of the totala+b−b−tilt pattern found in the ground-state structure, that is, described by the combination. The inset depicts the 100% rotational distortions. (d) Change in the position of the Sr and Ca conduction band centre of mass () and (e) variation in the number of states at the Fermi level [ΔN(EF)] normalized to the value without the polar distortion. The ferromagnetic state is stable for polar displacements larger than ~0.25 Å. 1 and Supplementary Table 4 ). Note that the hypothetical structure would be related to an experimentally accessible high-temperature phase, assuming that the crystal would not first decompose. The normalized distortion vector is , where corresponds to a polar ir -active mode, and and describe k ≠0 in-phase and out-of-phase rotation modes, respectively. The amplitude and energetic contribution of each irrep in the polar structure provide insight into the stability of the NSCM ( Fig. 4 ). Although the zone-centre polar mode transforming as irrep is weakly unstable in the high-symmetry P 4/ mmm structure (see Supplementary Fig. 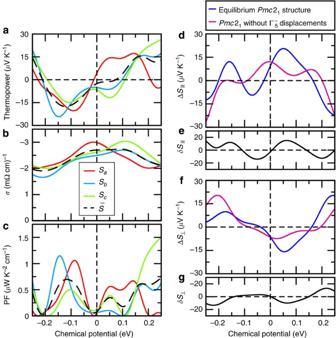Figure 5: Chemical potential-dependent properties and anisotropy at 300 K. (Sr,Ca)Ru2O6transport properties (left panels) as a function of the chemical potentialμ: (a) thermopowerS, (b) conductivityσand (c) the power factor PF. Red, blue and green lines are the transport properties along thea,band the polarcaxis, respectively. The dashed line indicates the total behaviour, given as an average of the three principle components. Anisotropy (right panels) along (d) theabplane (ΔS||) with (blue) and without (magenta) polar displacements; the difference of the two curves is depicted in (e). (f) The anisotropy between the polarcaxis and theabplane (ΔS⊥), and (g) the difference between the two curves. 2 and Supplementary Table 5 ), that is, characterized by a negative quadratic energy surface with respect to the increasing amplitude of the polar distortion ( Fig. 4a ), its energetic contribution to the ground state structure is two orders of magnitude smaller than that obtained from the octahedral rotation modes ( Fig. 4b ). To show that the geometric RuO 6 rotations drive the polar Sr and Ca displacements ( Fig. 4 a, inset), circumventing the contraindication between metallicity and the ir -mode, we map the total energy evolution of (Sr,Ca)Ru 2 O 6 with increasing amplitude of the ir -polar mode at different fixed values of the a + b − b − tilt pattern described by ( ) ( Fig. 4c ). We find that with increasing amplitude of the a + b − b − tilt pattern, the negative curvature about the origin vanishes; the energy landscape evolves to a parabola with a single energy minimum, indicating the hardening (stabilization) of the polar phonon mode at finite amplitude induced by the geometric RuO 6 octahedral rotations, which fully accounts for the loss of inversion symmetry. Figure 4: Electron–lattice interactions on the ground state stability. ( a ) Polar ( ir -active) mode with symmetry. The inset depicts the polar cation displacement pattern; apical oxygen and (small) Ru displacements are omitted for clarity. ( b ) In-phase and out-of-phase RuO 6 rotational modes. ( c ) Normalized energy gain obtained by increasing amplitude of the polar displacements at fixed percentages of the total a + b − b − tilt pattern found in the ground-state structure, that is, described by the combination . The inset depicts the 100% rotational distortions. ( d ) Change in the position of the Sr and Ca conduction band centre of mass ( ) and ( e ) variation in the number of states at the Fermi level [Δ N ( E F )] normalized to the value without the polar distortion. The ferromagnetic state is stable for polar displacements larger than ~0.25 Å. Full size image Figure 4d shows there are minor changes in the position of the band centre of mass for the principal atoms involved in the polar mode, that is, the Ca (4 s 3 d ) and Sr (5 s 4 d ) states, which are located ~6.2 eV above E F in the conduction band. The relative change in the number of states at the Fermi level (Δ N ( E F ), Fig. 4e ) is also small with respect to the centrosymmetric structure and increasing amplitude of the polar mode, confirming the weak interaction between the inversion symmetry-lifting displacements and the low-energy electronic structure. The conduction bands marginally shift to higher energy (~0.06 eV) and the change in N ( E F ) is ~±5%, validating the proposed NCSM design guidelines. Interestingly, the polar mode activates the ferromagnetic ground state observed by the exchange split electronic structure that appears around ~0.25 Å in Fig. 4e , indicative of large spin–phonon coupling [38] , [39] . Thermoelectric response Owing to the orthorhombicity in (Sr,Ca)Ru 2 O 6 , the recent interest in thermoelectric properties of perovskite oxide superlattices [40] , and the fact that degenerately doped ferroelectrics with polar axes exhibit unusual thermoelectric properties [41] , [42] , [43] , we evaluate the thermopower anisotropy at 300 K using Botlzmann transport theory within the constant scattering time approximation. Figure 5 shows the relevant thermoelectric properties in the chemical potential range varying from −0.25 to 0.25 eV. The average thermopower , denoted by the broken line in Fig. 5a , ranges from 14 to −18 μ V K −1 with two sign changes near μ ≃ −0.21 and μ ≃ 0.07 eV, indicating a change in the dominant charge carriers from holes to electrons and then from electrons to holes, respectively. We also note that above μ ≃ 0.16 eV, the thermopower components along the polar c direction dominate the thermal properties. Figure 5: Chemical potential-dependent properties and anisotropy at 300 K. (Sr,Ca)Ru 2 O 6 transport properties (left panels) as a function of the chemical potential μ : (a) thermopower S , (b) conductivity σ and ( c ) the power factor PF. Red, blue and green lines are the transport properties along the a , b and the polar c axis, respectively. The dashed line indicates the total behaviour, given as an average of the three principle components. Anisotropy (right panels) along ( d ) the ab plane (Δ S || ) with (blue) and without (magenta) polar displacements; the difference of the two curves is depicted in ( e ). ( f ) The anisotropy between the polar c axis and the ab plane (Δ S ⊥ ), and ( g ) the difference between the two curves. Full size image The conductivity σ is found to oscillate in a narrow window over the chemical potential range considered, and all the three components resolved along the crystallographic axes exhibit similar behaviour ( Fig. 5b ). Above μ ≃ 0.05 eV, where the Seebeck coefficient along the polar axis is extremized, the conductivity along the c axis ( σ c ) begins to exceed that along the other directions. Figure 5c shows the total and crystal axis-decomposed power factor PF= σS 2 . The total power factor exhibits a pronounced local maximum, PF ≃ 0.7 μ W K −2 cm −1 , near μ =−0.12 eV (hole doping h =3 × 10 21 cm −3 ), and two other less pronounced local maxima, PF ≃ 0.35 μ W K −2 cm −1 at μ ~0.05 eV and μ ~0.18 eV, which are negligible when compared with thermoelectric materials found in applications (20–50 μ W K −2 cm −1 ) [44] . It is interesting, however, that the maximum at μ ~0.18 eV (electron doping of n =6 × 10 21 cm −3 ) is in the region where the Seebeck coefficient and the conductivity along the polar axis both dominate the transport behaviour along the other directions. To show that this anisotropy arises from the polar displacements and not the orthorhombic lattice symmetry of (Sr,Ca)Ru 2 O 6 , we calculate the thermopower anisotropy in the ab plane as ( Fig. 5d ), and the thermopower anisotropy along the polar c axis as ( Fig. 5f ), for the equilibrium Pmc 2 1 structure and for a hypothetical structure with the polar atomic displacements described by irrep fully removed. When we remove the polar displacements, we find that Δ S || is modified for all chemical potentials examined, except at 0 eV. The difference between the two cases Δ S || ranges between ±15 μ V K −1 ( Fig. 5e ). The thermopower anisotropy along the polar c axis, Δ S ⊥ , behaves as Δ S || , except for a sign change at 0 eV: The difference in the c axis anisotropy, δ S ⊥ , also ranges between ±15 μ V K −1 for the two structures ( Fig. 5g ). Consistent with our design guidelines, at μ =0 eV, the change in the thermopower anisotropy is essentially zero, indicating weak coupling between the states at the Fermi level and the polar atomic displacements that lift inversion symmetry. The role of the polar distortions becomes even more evident by analysing the anisotropy change in the bc plane (see Supplementary Fig. 3 ) where the lattice parameters are identical. The removal of polar displacements is found to produce a shift relative to the chemical potential below μ =0.18 eV. Above this value, we find that the anisotropy in the bc plane is small in the structure without the polar distortions, whereas it is maximized in the equilibrium structure. Such behaviour is also observed in Fig. 5f over the same electron-doped region. The magnitude of the anisotropy, |δ S ⊥ |, in the ground state structure exceeds that of the phase with the polar displacements removed. 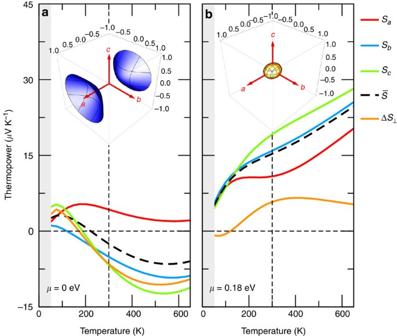Figure 6: Temperature-dependent thermopower in paramagnetic (Sr,Ca)Ru2O6. Temperature-dependent thermopower along thea,bandcaxes at (a)μ=0 eV and (b)μ=0.18 eV. The shaded area indicates the ferromagnetic phase below the calculated Curie temperatureTc~50 K. The average thermopower is calculated as. The insets depict the 300 K quadric surface representations of the second-rank Seebeck tensor, revealing enhanced anisotropy on doping along the polar axis. Figure 6 shows the computed temperature-dependent thermopower S as a function of chemical potential μ =0 and 0.18 eV, which is selected because the power factor ( σS 2 ) exhibits a local maximum that is due mainly to the Seebeck coefficient along the polar axis, S c ( Fig. 5c ). Due to identical lattice constants along the b and c axes in (Sr,Ca)Ru 2 O 6 , S b and S c have similar behaviour for μ =0 eV. The total thermopower, , ranges from ~2.5 to −7 μ V K −1 and exhibits parabolic behaviour with a maximum around 550 K. The thermopower anisotropy along the polar c axis, Δ S ⊥ , exhibits the same behaviour. At μ =0 eV, the thermopower anisotropy is relatively large (|Δ S ⊥ |~6.3 μ V K −1 ), reflected in the 300 K representation of the second-rank Seebeck tensor (inset) appearing as a hyperboloid with two sheets. Figure 6: Temperature-dependent thermopower in paramagnetic (Sr,Ca)Ru 2 O 6 . Temperature-dependent thermopower along the a , b and c axes at ( a ) μ =0 eV and ( b ) μ =0.18 eV. The shaded area indicates the ferromagnetic phase below the calculated Curie temperature T c ~50 K. The average thermopower is calculated as . The insets depict the 300 K quadric surface representations of the second-rank Seebeck tensor, revealing enhanced anisotropy on doping along the polar axis. Full size image For μ =0.18 eV the scenario is different. has a quasi-linear behaviour from low to high temperature: S a , S b and S c all become positive. Over the entire temperature range considered, the thermopower along the polar axis S c dominates. At 300 K (broken vertical line), the second-rank Seebeck tensor quadric surface becomes an elongated ellipsoid, flattened along the c direction. Accordingly the thermopower anisotropy at 300 K becomes ~5.8 μ V K −1 . The thermoelectric behaviour as a function of doping can be understood by examining the electronic band structures of the equilibrium Pmc 2 1 structure with that of the hypothetical (Sr,Ca)Ru 2 O 6 system with the polar atomic displacements removed ( Fig. 7 ). Inspection of the electronic band structure along the lines of symmetry X – S (corresponding to b in real space) and S – R (corresponding to the polar c axis) reveals strongly hybridized Ru 4 d –O 2 p bands dispersing from −0.2 eV to 0.3 eV, where the electron contribution dominates until ~0.07 eV above the Fermi level ( Fig. 7a ), explaining the sign change of near μ ≃ 0.07 eV in Fig. 5a . 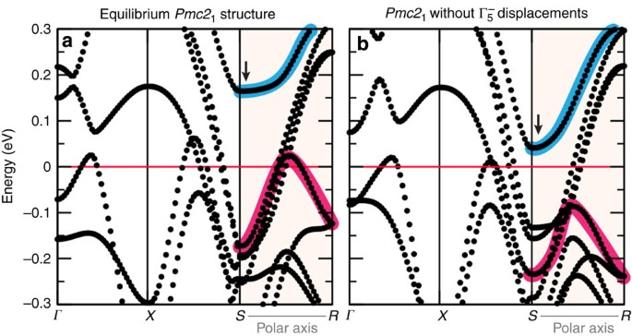Figure 7: Effect of polar displacements on the electronic structure. In the left (right) panel the bands structure for the non-magnetic layered (Sr,Ca)Ru2O6(withoutdisplacements). The highlighted bands are mainly affected by the polar displacements. The red (lower energy) bands are partially occupied in the equilibrium structure. The shaded path corresponds to ak-space trajectory parallel to the polar axis. Brillouin zone labels:Γ(0, 0, 0),X(π/2, 0, 0),S(π/2, π/2, 0),R(π/2,π/2,π/2). Figure 7: Effect of polar displacements on the electronic structure. In the left (right) panel the bands structure for the non-magnetic layered (Sr,Ca)Ru 2 O 6 (without displacements). The highlighted bands are mainly affected by the polar displacements. The red (lower energy) bands are partially occupied in the equilibrium structure. The shaded path corresponds to a k -space trajectory parallel to the polar axis. Brillouin zone labels: Γ (0, 0, 0), X ( π /2, 0, 0), S ( π /2, π/2, 0), R ( π /2, π /2, π /2). Full size image In addition, the polar displacements largely modify the band structure along S − R in the energy range 0.05–0.30 eV. In the absence of the polar mode, the band near 0.16 eV (arrow in Fig. 7 ), which is derived from the oxygen 2 p states in the CaO and SrO planes, shifts to lower energy and broadens. In the equilibrium structure, this band along S – R is higher in energy than the band which changes dispersion along Γ – X (energy range 0.05–0.18 eV); however, when the polar displacements are removed, the oxygen-derived band along S – R becomes lower than that of the band centre of mass along Γ – X . It is the dependence of these two bands on the amplitude of the polar atomic displacements that leads to the different behaviour appearing in Fig. 5f for μ =0.18 eV. We find that the 300 K thermopower anisotropy of (Sr,Ca)Ru 2 O 6 is close to that of centrosymmetric YBa 2 Cu 3 O 7− δ (YBCO, ~7–10 μ V K −1 ) [45] , [46] , which exhibits strong thermal and electrical anisotropy owing to the two-dimensional (2D) crystal structure. The thermopower anisotropy in other metallic systems, for example, the hexagonal delafossite oxides PdCoO 2 and PtCoO 2 (ref. 47 ), also derive from the 2D layered topology of the system, and so present large Seebeck coefficients along the trigonal axis, that is, the axis which is most insulating. In contrast, the thermopower anisotropy in (Sr,Ca)Ru 2 O 6 is not related to the dimensionality of the system, but rather to the existence of a polar axis along which the electrical conductivity is highest. The peculiar thermopower anisotropy in (Sr,Ca)Ru 2 O 6 dictates that the electric field resulting from an applied heat flux to the material will be non-collinear. This property is a fundamental feature for any anisotropic thermoelectric devices [48] . It enables the heat flux to be measured in a geometry perpendicular to the induced electrical current, specifically at locations where the temperatures are equal (see Supplementary Fig. 4 and Supplementary Note 1 ). Given the metallic conductivity of (Sr,Ca)Ru 2 O 6 and that the relaxation time is small in comparison with that of semiconductors or insulators already finding use in thermoelectric devices, this polar NCSM would enable sensing on sub-nanosecond timescales (comparable to YBCO [46] ). New applications of these oxide materials could be found in ultrafast thermoelectric devices [46] , [48] , where stability under extreme conditions, speed, and the ability to measure heat fluxes of high density are key requirements, for example, thermal (heat) radiation detectors. Moreover, because of the compatibility of perovskite oxides with Si-based CMOS technologies [49] , we anticipate that these designed NCSMs will more readily find integration and device development than previously identified materials with large anisotropic thermoelectric responses. In summary, we designed a polar noncentrosymmetric ruthenate conductor and described how to eliminate the incompatibility between metallicity and acentricity in complex transition metal oxides. We articulated a paradigm for which new NCMS may be found, and showed that (Sr,Ca)Ru 2 O 6 exhibits Seebeck coefficients with anisotropy derived from the polar structure. We believe that other polar metals could exhibit such anisotropic thermal properties; the important discriminating feature, however, is the k -space evolution of the electronic structure with the real space polar distortion. Broadly, such thermopower anisotropy may also be found in any NCSM, for example, in compounds which are chiral but non-polar, but continued studies are required to clarify the extent of the response. We hope this work motivates the synthesis of new materials and the discussion of new applications where highly anisotropic thermoelectric responses in metals can be leveraged. Ab initio calculations and group theoretical analysis We perform first-principles density functional calculations within the local spin density approximation, which is known to provide a reliable description of perovskite ruthenates [35] , [39] , [50] as implemented in the Vienna Ab initio Simulation Package [51] , [52] . Calculations carried out with the Perdew–Burke–Ernzerhof generalized gradient approximation functional revised for solids [53] provide essentially the same results (see Supplementary Table 6 ). We use the projector augmented wave method [54] to treat the core and valence electrons using a 550 eV plane wave expansion and the following electronic configurations: 4 s 2 4 p 6 5 s 2 (Sr), 3 p 6 4 s 2 (Ca), 4 p 6 5 s 2 4 d 6 (Ru) and 2 s 2 2 p 4 (O). A 7 × 7 × 5 Monkhorst-Pack k -point mesh [55] and Gaussian smearing (20 meV width) was used for the Brillouin zone (BZ) sampling and integrations. For structure optimization, we relax the atomic positions to have forces less than 0.1 meV Å −1 . We impose as a constraint b = c (note that in bulk ruthenates the deviations between the ‘short’ axes are small [39] ) to simulate the situation under thin-film growth on a cubic substrate with a square lattice net. We search for the ground state structure by computing the phonon frequencies and eigenmodes of the high-symmetry centrosymmetric (Sr,Ca)Ru 2 O 6 structure (space group P 4/ mmm ), and then systematically ‘freeze-in’ linear combinations of the unstable modes, performing structural optimization on these candidate low-symmetry structures until the global minimum is obtained. The group theoretical analysis was aided with the ISODISTORT [56] and AMPLIMODES [57] , [58] software. Thermoelectric properties For the calculation of the Seebeck coefficient and other transport properties, we use Boltzmann transport theory [59] within the constant scattering time ( τ ) approximation as implemented in the boltztrap code [61] . We perform a non-self-consistent band-structure calculation with a much denser sampling of 27 × 33 × 33 (4,046 k -points in the irreducible BZ; 29,403 k -points in the full BZ), using the equilibrium ground state structure. The Seebeck coefficients S are calculated independently from τ . The electrical conductivity, however, requires a known value of τ , and so we introduce an empirical parameter. Here, the relaxation time value τ =0.23 × 10 −14 s is employed in all calculations, which we obtain from fitting the room-temperature conductivity [62] σ ~2.7 × 10 5 S m −1 of solid solution Sr 0.5 Ca 0.5 RuO 3 . We believe this estimate to provide a meaningful approximation based on our excellent agreement with other physical properties of the solid solution reported in the main text. The thermoelectric properties at room temperature are calculated using the zero-Kelvin polar structure based on the fact that the high-temperature structural transitions away from orthorhombic symmetry in bulk CaRuO 3 and SrRuO 3 do not occur until 1,550 K [63] and 685 K, respectively [64] . On the basis of our calculated magnetic Curie temperatures of ~50 K, we also compute all thermoelectric responses using a non-magnetic configuration. How to cite this article: Puggioni, D. et al. Designing a robustly metallic noncenstrosymmetric ruthenate oxide with large thermopower anisotropy. Nat. Commun. 5:3432 doi: 10.1038/ncomms4432 (2014).